Activation of TREK-1 by morphine results in analgesia without adverse side effects Morphine is the gold-standard pain reliever for severe acute or chronic pain but it also produces adverse side effects that can alter the quality of life of patients and, in some rare cases, jeopardize the vital prognosis. Morphine elicits both therapeutic and adverse effects primarily through the same μ opioid receptor subtype, which makes it difficult to separate the two types of effects. Here we show that beneficial and deleterious effects of morphine are mediated through different signalling pathways downstream from μ opioid receptor. We demonstrate that the TREK-1 K + channel is a crucial contributor of morphine-induced analgesia in mice, while it is not involved in morphine-induced constipation, respiratory depression and dependence—three main adverse effects of opioid analgesic therapy. These observations suggest that direct activation of the TREK-1 K + channel, acting downstream from the μ opioid receptor, might have strong analgesic effects without opioid-like adverse effects. Most opioid analgesic drugs, such as morphine, modulate nociception by stimulating the G-protein-coupled μ opioid receptors (μORs), the major molecular gate for opioid analgesia [1] . It is well documented that neither the analgesic nor adverse pharmacological activities of morphine can be detected in mutant mice lacking μOR [2] . This explains the difficulty in separating the beneficial and adverse effects of μOR agonists. Pharmacological studies have long suggested the existence of different subtypes of μOR, and the possibility of dissociating analgesia from several opioid adverse effects [3] , [4] , [5] , yet without success. Recently, truncated μOR splice variants [6] have also been proposed as targets to improve benefit/risk ratio of opiate analgesics [7] . Several other strategies have been developed to try to reduce opioids’ adverse effects, such as the use of either agonists of other opioid receptors [8] , [9] or peripheral μOR antagonists (for example, methynaltrexone [10] and alvimopan [11] ). However, the former ones produce a limited analgesia [12] and the latter ones need to be co-prescribed with opioids and prevent constipation but not morphine central adverse effects such as respiratory depression [13] . Alternatively, a better comprehension of signalling pathways and downstream effectors from μOR that are potentially involved in opiates’ analgesic effects would facilitate finding new targets for analgesic compounds with higher benefit/risk ratio. Although not completely understood, binding of morphine to μOR results in the activation of a G i/o protein, inhibition of adenylate cyclase and activation of phospholipase C, and consequently, inhibition of voltage-dependent Ca 2+ channels as well as activation of K + channels [14] . G protein-activated inwardly rectifying K + (GIRK) channels were considered as prominent K + channels in opioid-induced analgesia [15] . However, studies using the GIRK-channel inhibitor tertiapine [16] , or GIRK knockout (KO) mice [16] , [17] , demonstrated only a partial role for these channels in the antinociceptive effect mediated by high doses of morphine. The TREK-1 channel is a member of the two-pore domain K + (K 2P ) channel family with background activity [18] . It is expressed in sensory neurons, particularly in nociceptors [19] , and is also broadly distributed in the central nervous system [18] . We have previously demonstrated the role of this channel in polymodal pain perception [19] , [20] . Moreover, recent data have shown an enhancement of TREK-1 activity in response to the activation of G α i -coupled receptors [21] , [22] . Consequently, we evaluated the implication of the TREK-1 channel in the antinociceptive effect and in the main adverse effects of morphine using TREK-1 KO mice and their wild-type littermates. In this study, we show the major involvement of the TREK-1 channel as an effector of μOR in the analgesic effect of morphine. Interestingly, we also observe that this channel is not involved in usual adverse effects of morphine such as constipation, respiratory depression and dependence. These observations suggest that direct activation of the TREK-1 channel, acting downstream from the μOR, might have strong analgesic effects without opioids-like adverse effects. The analgesic effect of morphine involves TREK-1 The analgesic effect of morphine was assessed using thermal nocifensive pain tests. First, in accordance with previous results [19] , we observed that TREK-1 −/− mice demonstrated a higher sensitivity as compared with wild-type mice in the tail immersion test at 46 °C (see Supplementary Fig. S1a ), whereas no difference was observed in the hot-plate test at 52 °C (see Supplementary Fig. S1b ). We then assessed, in naive mice, the involvement of TREK-1 in the antinociceptive effect of morphine by measuring the withdrawal latencies at both temperatures. The effect of morphine was determined by calculating the variation between pretreatment and post-treatment latencies for each animal. The assessment of the kinetics of the antinociceptive effect of systemic administrations of increasing doses of morphine (1, 3 and 5 mg kg −1 , subcutaneous (s.c.)) demonstrated a significant decrease in analgesia in TREK-1 −/− mice compared with their TREK-1 +/+ littermates in the two tests (areas under the time course curves were decreased: −40.3% and −47.1% in the tail immersion test at 3 and 5 mg kg −1 of morphine, respectively; −66.0% and −59.7% in the hot-plate test, respectively) ( Fig. 1a,b right panels). This decrease was confirmed when comparing both scores at the peak effect ( Fig. 1a,b left panels) and by another experiment using 1, 3, 5, 10 and 20 mg kg −1 of morphine, in which the mean (±s.e.m.) ED50 values in the tail immersion test were 13.3±1.1 and 9.2±0.6 mg kg −1 in TREK-1 −/− mice and their TREK-1 +/+ littermates, respectively ( n =10 per dose). Furthermore, this study shows a more important contribution of TREK-1 deletion in morphine analgesia for the lowest doses: 55, 58, 35 and 21% for 3, 5, 10 and 20 mg kg −1 , respectively (see day 1 scores in Fig. 2b,c ). Taken together, these results demonstrate that TREK-1 is a major effector of morphine-induced thermal analgesia. Similarly, there was a strong reduction (−80.0%) in the analgesic activity of fentanyl (0.03 mg kg −1 , s.c.), a μOR selective agonist, in TREK-1 −/− mice ( Supplementary Fig. S2 ). Interestingly, intrathecally administered tertiapin, a GIRK-channel inhibitor, partially decreased the antinociceptive effect of a high dose of morphine (5 mg kg −1 , s.c.) but did not affect the antinociceptive effect of 3 mg kg −1 of morphine ( Supplementary Fig. S3 ). 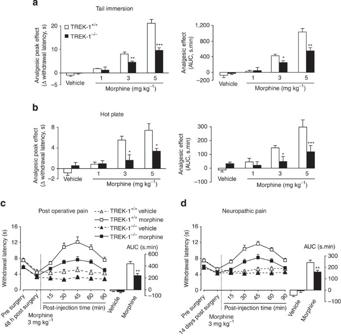Figure 1: Involvement of the TREK-1 channel in morphine-induced analgesia. (a,b) Antinociceptive effect of systemic administration of morphine in healthy wild-type andTREK-1−/−mice littermates assessed by the tail immersion test (46 °C) (a) or the hot-plate test (52 °C) (b). Mice were injected either with morphine (1, 3 or 5 mg kg−1, s.c.) or saline. Pre- and post- (15, 30, 45, 60 and 90 min after) treatment withdrawal latencies were assessed. For the two parts, (a,b), data are represented, on the right panels, as the mean±s.e.m. of the areas under the time course curves (AUC, s.min) of analgesia scores (differences between post- and pretreatment withdrawal latencies) and, on the left panels, as the mean±s.e.m of the peak effect 30 min after injection.n=8–10 per dose for each genotype. A significant decrease in systemic morphine-induced analgesia was observed in healthyTREK-1−/−mice as compared withTREK-1+/+animals. (c,d) Antihyperalgesic effect of systemic administration of morphine in wild-type andTREK-1−/−mice assessed by the paw immersion test (46 °C) following induction of a postoperative pain model (plantar skin and muscle incision) (c) or a neuropathic pain model (chronic constriction injury of the sciatic nerve) (d). Baseline latencies were recorded before surgery and the antihyperalgesic effect of morphine was assessed 48 h and 14 days after surgery for postoperative pain and neuropathic pain models, respectively. Mice were injected either with morphine (3 mg kg−1, s.c.) or saline. Pre- and post- (15, 30, 45, 60 and 90 min after) treatment, pain thresholds were assessed. Data forc,drepresent mean±s.e.m. The inset shows the mean±s.e.m. of AUC of analgesia scores (differences between post- and pretreatment withdrawal latencies).n=8–10 per dose for each genotype. A significant decrease in morphine-induced antihyperalgesia was observed inTREK-1−/−mice as compared withTREK-1+/+animals. Statistical analysis was performed using two-way ANOVA followed by Student–Newman–Keulspost-hoctest; *P<0.05, **P<0.01,***P<0.001,TREK-1+/+versusTREK-1−/−. Figure 1: Involvement of the TREK-1 channel in morphine-induced analgesia. ( a , b ) Antinociceptive effect of systemic administration of morphine in healthy wild-type and TREK-1 −/− mice littermates assessed by the tail immersion test (46 °C) ( a ) or the hot-plate test (52 °C) ( b ). Mice were injected either with morphine (1, 3 or 5 mg kg −1 , s.c.) or saline. Pre- and post- (15, 30, 45, 60 and 90 min after) treatment withdrawal latencies were assessed. For the two parts, ( a , b ), data are represented, on the right panels, as the mean±s.e.m. of the areas under the time course curves (AUC, s.min) of analgesia scores (differences between post- and pretreatment withdrawal latencies) and, on the left panels, as the mean±s.e.m of the peak effect 30 min after injection. n =8–10 per dose for each genotype. A significant decrease in systemic morphine-induced analgesia was observed in healthy TREK-1 −/− mice as compared with TREK-1 +/+ animals. ( c , d ) Antihyperalgesic effect of systemic administration of morphine in wild-type and TREK-1 −/− mice assessed by the paw immersion test (46 °C) following induction of a postoperative pain model (plantar skin and muscle incision) ( c ) or a neuropathic pain model (chronic constriction injury of the sciatic nerve) ( d ). Baseline latencies were recorded before surgery and the antihyperalgesic effect of morphine was assessed 48 h and 14 days after surgery for postoperative pain and neuropathic pain models, respectively. Mice were injected either with morphine (3 mg kg −1 , s.c.) or saline. Pre- and post- (15, 30, 45, 60 and 90 min after) treatment, pain thresholds were assessed. Data for c , d represent mean±s.e.m. The inset shows the mean±s.e.m. of AUC of analgesia scores (differences between post- and pretreatment withdrawal latencies). n =8–10 per dose for each genotype. A significant decrease in morphine-induced antihyperalgesia was observed in TREK-1 −/− mice as compared with TREK-1 +/+ animals. Statistical analysis was performed using two-way ANOVA followed by Student–Newman–Keuls post-hoc test; * P <0.05, ** P <0.01, *** P <0.001, TREK-1 +/+ versus TREK-1 −/− . 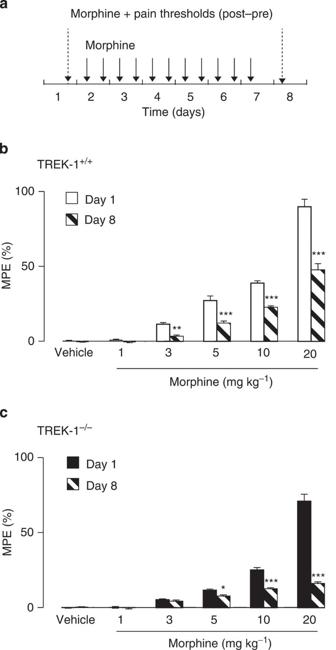Figure 2: Involvement of the TREK-1 channel in morphine-induced tolerance to analgesia. Degree of tolerance, represented by the loss of morphine-induced analgesic effect inTREK- 1+/+andTREK-1−/−mice after a 6-day treatment in the tail immersion test (46 °C). Comparison of morphine-induced analgesia (1, 3, 5, 10 or 20 mg kg−1, s.c.) or saline effect before (day 1) and after (day 8) a repeated morphine treatment (10 mg kg−1, s.c., twice a day on days 2–6 and once on day 7) (a) inTREK-1+/+mice (b) and inTREK-1−/−mice (c). Data are represented as mean±s.e.m. of percentage of the maximal possible effect (MPE)=100 × ((test withdrawal latency−baseline latency)/(cutoff−baseline latency)).n=12–13 per dose for each genotype. Statistical analysis was performed using two-way ANOVA followed by Student–Newman–Keulspost-hoctest; *P<0.05, **P<0.01, ***P<0.001, day 1 versus day 8 for (b,c). Full size image Figure 2: Involvement of the TREK-1 channel in morphine-induced tolerance to analgesia. Degree of tolerance, represented by the loss of morphine-induced analgesic effect in TREK- 1 +/+ and TREK-1 −/− mice after a 6-day treatment in the tail immersion test (46 °C). Comparison of morphine-induced analgesia (1, 3, 5, 10 or 20 mg kg −1 , s.c.) or saline effect before (day 1) and after (day 8) a repeated morphine treatment (10 mg kg −1 , s.c., twice a day on days 2–6 and once on day 7) ( a ) in TREK-1 +/+ mice ( b ) and in TREK-1 −/− mice ( c ). Data are represented as mean±s.e.m. of percentage of the maximal possible effect (MPE)=100 × ((test withdrawal latency−baseline latency)/(cutoff−baseline latency)). n =12–13 per dose for each genotype. Statistical analysis was performed using two-way ANOVA followed by Student–Newman–Keuls post-hoc test; * P <0.05, ** P <0.01, *** P <0.001, day 1 versus day 8 for ( b , c ). Full size image Since morphine is used to treat severe acute and chronic pain in humans [23] , such as postoperative pain and, in some cases, neuropathic pain, we investigated the role of TREK-1 channels in pathological pain models. We tested the antihyperalgesic effect of morphine in a post-surgical pain model induced by a plantar incision of the mouse left hindpaw [24] and in a neuropathic pain model following chronic constriction injury by ligature of the left sciatic nerve [25] . Areas under the time course curves of morphine (3 mg kg −1 , s.c.)-induced antihyperalgesia were strongly reduced in TREK-1 −/− mice compared with TREK-1 +/+ littermates in the paw immersion test at 46 °C, 48 h post surgery (−44.6%) and 14 days after chronic constriction injury (−34.6%) ( Fig. 1c,d , respectively). These results clearly demonstrate that TREK-1 is a downstream effector of μOR involved in morphine-induced analgesia. Tolerance to morphine is a phenomenon closely linked to its analgesic effect as it corresponds to a reduction of its effect after a prolonged exposure. A prolonged 6-day treatment of two daily injections of high doses of morphine (cumulative dose of 130 mg kg −1 , s.c.) ( Fig. 2a ) significantly decreased the analgesic potency of a single dose of morphine (3, 5, 10 or 20 mg kg −1 , s.c.) in TREK-1 +/+ mice (−72.6%, −56.1%, −41.9% and −51.2%, respectively) ( Fig. 2b ), while this tolerance did not appear in the absence of the channel, in TREK-1 −/− mice for the dose of 3 mg kg −1 (s.c.) of morphine. In this genotype, a small degree of tolerance was observed at 5 mg kg −1 (s.c.) (−34.8%), while it increased for higher doses (−50.6% and −77.5% for 10 and 20 mg kg −1 , s.c., respectively) and became not statistically different from that observed in littermates ( Fig. 2c ). This is further evidence of an important contribution of the TREK-1 channel to the analgesic effect of morphine, especially at doses up to 5 mg kg −1 (s.c.), which are commonly used to assess the analgesic effect of morphine. We confirm, using electrophysiology (patch-clamp) technique, that a functional coupling exists between μOR and the TREK-1 channel. When the two proteins were co-expressed in COS cells, morphine activated the TREK-1 channel ( Fig. 3a,b ). Moreover, the functional coupling was lost with a serine 333 to aspartic acid mutant of the TREK-1 channel (TREK-1S333D) that mimics phosphorylation of the channel on the regulatory serine 333 by PKA and diminishes basal current [26] ( Fig. 3c,d ). Thus serine 333, the main amino acid of TREK-1 involved in PKA-dependent phosphorylation [22] , [27] , appears to be essential for the activation of the channel by morphine. 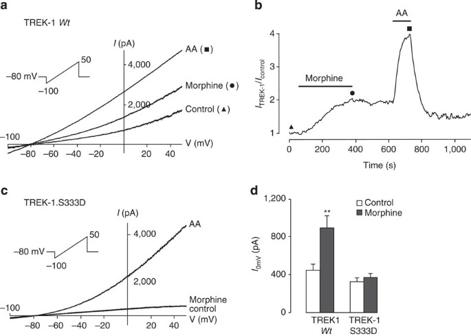Figure 3: Evidence of the functional coupling between μOR and TREK-1 in COS cells. (a), I–V curves of TREK-1 channels elicited by voltage ramps (−100 to +50 mV, 800 ms) applied every 20 s on COS cells expressing the wild-type TREK-1 channel, in presence of 10 μM morphine or 10 μM arachidonic acid (AA) acutely perfused on the cell, or in control condition. (b) Characteristic current trace showing the activation of TREK-1 current, measured at 0 mV, by perfusion of 10 μM morphine followed by 10 μM arachidonic acid. (c) I–V curves acquired on COS cells expressing the mutant TREK-1.S333D channel in presence of 10 μM morphine, 10 μM AA or in control condition. (d) Mean±s.e.m. of wild-type TREK-1 and TREK-1.S333D current intensity in presence of 10 μM morphine and in control condition, recorded at 0 mV. Morphine significantly increased wild-type TREK-1 current (n=10, **P<0.005, Wilcoxon matched pairs test) but had no effect on the mutant channel (n=6, Wilcoxon matched pairs test). Figure 3: Evidence of the functional coupling between μOR and TREK-1 in COS cells. ( a ), I–V curves of TREK-1 channels elicited by voltage ramps (−100 to +50 mV, 800 ms) applied every 20 s on COS cells expressing the wild-type TREK-1 channel, in presence of 10 μM morphine or 10 μM arachidonic acid (AA) acutely perfused on the cell, or in control condition. ( b ) Characteristic current trace showing the activation of TREK-1 current, measured at 0 mV, by perfusion of 10 μM morphine followed by 10 μM arachidonic acid. ( c ) I–V curves acquired on COS cells expressing the mutant TREK-1.S333D channel in presence of 10 μM morphine, 10 μM AA or in control condition. ( d ) Mean±s.e.m. of wild-type TREK-1 and TREK-1.S333D current intensity in presence of 10 μM morphine and in control condition, recorded at 0 mV. Morphine significantly increased wild-type TREK-1 current ( n =10, ** P <0.005, Wilcoxon matched pairs test) but had no effect on the mutant channel ( n =6, Wilcoxon matched pairs test). Full size image TREK-1 is not involved in morphine-induced adverse effects Constipation is the most usual complaint of patients treated with morphine [28] . We assessed the role of TREK-1 in the effect of morphine on gastrointestinal function by the quantification of fecal boli production in mice. To assure that both genotypes eat similarly, food consumption was monitored during 24 h for each mouse strain and expressed as grams of food ingested. No difference was observed between TREK-1-deficient mice and their wild-type littermates ( Supplementary Fig. S4 ). Morphine (1, 3 and 5 mg kg −1 , s.c.) induced a dose-dependent suppression of defecation in both groups of mice with no significant difference concerning the weight of stools collected over the 2-h period following the treatment with morphine ( Fig. 4a ). To further study the potential role of TREK-1 in the effect of morphine on gastrointestinal transit, we compared small intestinal transit times by following the progression of a methylene blue dye given by oral gavage. Morphine (1, 3 or 5 mg kg −1 , s.c.), administered 20 min before methylene blue ingestion, induced a dose-dependent reduction of the gastrointestinal transit ( Fig. 4b ) with no difference between genotypes, suggesting that TREK-1 does not interfere with the inhibitory effect of morphine on the motility of the small intestinal portion of the gastrointestinal tract. We next assessed whether morphine differentially affects colonic motility in TREK-1 −/− mice and TREK-1 +/+ littermates. Ex vivo recordings of isolated colon showed similar changes of migrating myoelectric complexes of the colonic muscular wall ( Fig. 4c,d ) in TREK-1 −/− and TREK-1 +/+ mice. Indeed, morphine (1 μM) similarly induced a disorganized motor activity in the proximal part of the colon, whereas it totally inhibited contractile activity in the intermediate and distal colon. Thus, while strongly involved in the analgesic effect of morphine, the TREK-1 channel appears not to be involved in this frequent adverse effect. 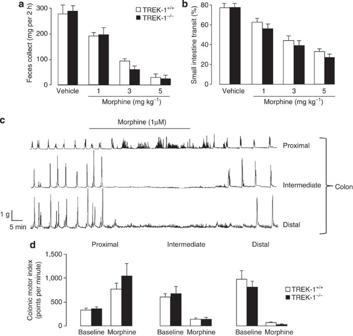Figure 4: Lack of involvement of the TREK-1 channel in morphine-induced constipation. (a) Evaluation of global fecal boli. Mice were treated with morphine (1, 3 or 5 mg kg−1, s.c.) or saline. Total defecation was weighed over a 2-h period after treatment. Data are represented as the mean±s.e.m.,n=8–9 per dose for each genotype. (b) Evaluation of gastrointestinal transit. Mice were treated with morphine (1, 3 or 5 mg kg−1, s.c.) or saline before they were orally given a solution of methylene blue. Mice were killed 30 min later and the percentage of small intestine stained, showing the distance travelled by the dye through the gastrointestinal tract, was measured. Data are represented as the mean±s.e.m.,n=8–9 per dose for each genotype. Statistical analysis was performed using two-way ANOVA,TREK-1+/+versusTREK-1−/−. (c,d)Ex vivoevaluation of morphine-induced constipation. (c) Example of migrating motor complexes (MMCs) recording in a colon isolated from aTREK-1+/+mouse. The circular muscle tensions recorded in the proximal, intermediate and distal zones of the colon, reflecting the spontaneous contractile activity, are shown. A 1-μM morphine perfusion disorganized the motor activity in the proximal part of the colon, whereas it totally inhibited the contractile activity of the intermediate and distal zones. (d) Comparative MMC index values obtained fromTREK-1+/+andTREK-1−/−mice in the proximal, intermediate and distal colon. After resampling the tension curves at 30 points per second, the number of points above the basal threshold value, considered as colonic contractile activity, was counted. Data are represented as the mean±s.e.m.,n=3–4 per genotype. Figure 4: Lack of involvement of the TREK-1 channel in morphine-induced constipation. ( a ) Evaluation of global fecal boli. Mice were treated with morphine (1, 3 or 5 mg kg −1 , s.c.) or saline. Total defecation was weighed over a 2-h period after treatment. Data are represented as the mean±s.e.m., n =8–9 per dose for each genotype. ( b ) Evaluation of gastrointestinal transit. Mice were treated with morphine (1, 3 or 5 mg kg −1 , s.c.) or saline before they were orally given a solution of methylene blue. Mice were killed 30 min later and the percentage of small intestine stained, showing the distance travelled by the dye through the gastrointestinal tract, was measured. Data are represented as the mean±s.e.m., n =8–9 per dose for each genotype. Statistical analysis was performed using two-way ANOVA, TREK-1 +/+ versus TREK-1 −/− . ( c , d ) Ex vivo evaluation of morphine-induced constipation. ( c ) Example of migrating motor complexes (MMCs) recording in a colon isolated from a TREK-1 +/+ mouse. The circular muscle tensions recorded in the proximal, intermediate and distal zones of the colon, reflecting the spontaneous contractile activity, are shown. A 1-μM morphine perfusion disorganized the motor activity in the proximal part of the colon, whereas it totally inhibited the contractile activity of the intermediate and distal zones. ( d ) Comparative MMC index values obtained from TREK-1 +/+ and TREK-1 −/− mice in the proximal, intermediate and distal colon. After resampling the tension curves at 30 points per second, the number of points above the basal threshold value, considered as colonic contractile activity, was counted. Data are represented as the mean±s.e.m., n =3–4 per genotype. Full size image Acute respiratory depression is a μOR-dependent adverse effect of morphine, which can have critical consequences as it may lead to death in the most severe cases. We analysed the breathing frequency of TREK-1 −/− mice and their wild-type littermates using whole-body plethysmography following administration of saline or high doses of morphine. Resting breathing frequency was not different between wild-type and TREK-1 −/− mice, and both saline and morphine (5 mg kg −1 ) treatments did not alter breathing frequency in either genotype ( Fig. 5 ). Whatever the genotype, morphine administration at higher doses of 10, 20 or 50 mg kg −1 s.c., largely above analgesic doses, induced a progressive and severe decrease in the respiratory rate ( Fig. 5 ) with the same intensity in the TREK-1 −/− and TREK-1 +/+ mice, which excludes an involvement of TREK-1 in this adverse effect. 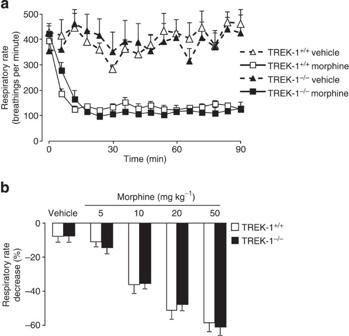Figure 5: Lack of involvement of the TREK-1 channel in morphine-induced respiratory depression. Evaluation of morphine-induced respiratory depression. (a) Respiratory rate curves ofTREK-1+/+andTREK-1−/−mice following administration of morphine (50 mg kg−1, s.c.) or saline. (b) Percentage of respiratory rate decrease inTREK-1+/+andTREK-1−/−mice following administration of morphine (5, 10, 20 or 50 mg kg−1, s.c.) or saline. Data are represented as the mean±s.e.m.,n=5–12 per dose for each genotype. Statistical analysis was performed using two-way ANOVA,TREK-1+/+versusTREK-1−/−. Figure 5: Lack of involvement of the TREK-1 channel in morphine-induced respiratory depression. Evaluation of morphine-induced respiratory depression. ( a ) Respiratory rate curves of TREK-1 +/+ and TREK-1 −/− mice following administration of morphine (50 mg kg −1 , s.c.) or saline. ( b ) Percentage of respiratory rate decrease in TREK-1 +/+ and TREK-1 −/− mice following administration of morphine (5, 10, 20 or 50 mg kg −1 , s.c.) or saline. Data are represented as the mean±s.e.m., n =5–12 per dose for each genotype. Statistical analysis was performed using two-way ANOVA, TREK-1 +/+ versus TREK-1 −/− . Full size image Chronic administration of morphine can also induce dependence with typical withdrawal symptoms when treatment is discontinued [29] . In humans, several signs such as anxiety, agitation and insomnia are observed. In mice, it is possible to assess this adverse effect through naloxone-precipitated withdrawal syndrome. Mice were injected twice a day for 6 days with high doses of morphine (cumulative dose of 130 mg kg −1 , s.c.) and, on day 7, a withdrawal syndrome was induced by a single injection of the non-selective opioid receptor antagonist naloxone (2 mg kg −1 , intraperitoneal (i.p.)) ( Fig. 6a ). No difference was observed between TREK-1 −/− and TREK-1 +/+ mice in scores of the assessed behavioural symptoms of morphine withdrawal—that is, the number of escape jumps, teeth chattering or paw tremour ( Fig. 6b–d ). 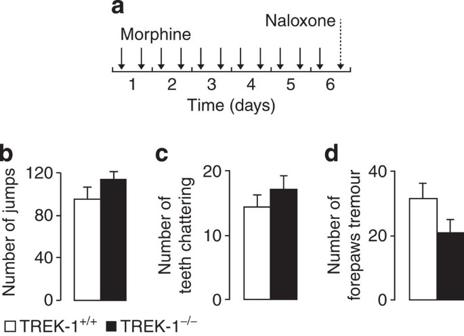Figure 6: Lack of involvement of the TREK-1 channel in morphine-induced dependence. Evaluation of morphine-induced dependence. Mice received repeated administrations of morphine over a 6-day period (10 mg kg−1, s.c., twice a day on days 1–5, once on day 6) and were subsequently treated with naloxone (2 mg kg−1, i.p.) on the last day (a). Behavioural response to withdrawal, characterized by jumps (b), teeth chattering (c) and forepaws tremor (d) were recorded over a 30-min period. Data are represented as the mean±s.e.m.,n=8–10 per dose for each genotype. Statistical analysis was performed using unpaired Student’st-test. Figure 6: Lack of involvement of the TREK-1 channel in morphine-induced dependence. Evaluation of morphine-induced dependence. Mice received repeated administrations of morphine over a 6-day period (10 mg kg −1 , s.c., twice a day on days 1–5, once on day 6) and were subsequently treated with naloxone (2 mg kg −1 , i.p.) on the last day ( a ). Behavioural response to withdrawal, characterized by jumps ( b ), teeth chattering ( c ) and forepaws tremor ( d ) were recorded over a 30-min period. Data are represented as the mean±s.e.m., n =8–10 per dose for each genotype. Statistical analysis was performed using unpaired Student’s t -test. Full size image In this study, we found that the background K + channel TREK-1 is involved in the analgesic effect of morphine but not in several adverse effects of this drug. Added to the known involvement of TREK-1 in the physiology of pain [19] , [20] , the present results thus suggest the great interest of TREK-1 as a target for new analgesic compounds with a good benefit/risk ratio. The TREK-1 channel appears to be a major contributor to the systemic morphine analgesic effect assessed both in acute pain tests and in models of pathological pain, which makes the demonstration of its involvement clinically relevant. Deletion of the TREK-1 channel results in a strong inhibition of the antinociceptive effect of morphine (3 mg kg −1 , s.c.) in both the tail immersion and the hot-plate tests (from 40% reduction of analgesic efficacy in the tail immersion test to 66% in the hot-plate test), confirmed by an increase of 45% of its ED50 in TREK-1 −/− mice compared with littermates. A similar reduction in the morphine analgesic effect was observed in pathophysiological models of post-surgical or neuropathic pain. This demonstrates that a functional link between μOR and the TREK-1 channel is needed for analgesia. TREK-1 involvement in morphine-induced antinociception occurs at lower analgesic doses than for GIRK channels. In comparison we found, in agreement with the literature [17] , that GIRK channels are only involved in the antinociceptive effect at higher doses of morphine (5 mg kg −1 ). Moreover, we demonstrate here that morphine-induced μOR activation leads to an increased TREK-1 current through PKA regulatory serine 333 in the C-terminal domain of the channel, as morphine-induced TREK-1 activation is suppressed when this amino acid is mutated. It is well documented that morphine reduces cAMP and PKA activities; thus, it can be proposed that morphine might alleviate the tonic PKA inactivation of TREK-1 channels, which would hyperpolarize the plasma membrane and depress neuronal activity in the pain pathway. A similar increase in TREK-1 current has been described with the activation of the G αi -coupled GPCR mGlu4 involving PKA phosphorylation on serine 333 (ref 21 ). Moreover, an increase in TREK-2 current, closely related to the TREK-1 channel, has been observed following activation of the G αi -coupled receptor GABA B . Baclofen, a GABA B agonist, has been shown to depress the adenylate cyclase/cAMP/PKA pathway and to reduce the tonic inhibition of PKA on TREK-2 channel, which reduced the excitability of stellate neurons by generating membrane hyperpolarization [30] . Interestingly, mGlu4 and GABA B agonists have been shown to possess an analgesic effect [31] , [32] , [33] , [34] . This interaction between morphine and TREK-1 is supposed to be located at the central level, as morphine is a centrally acting analgesic drug. At the spinal level, where morphine is known to act on the pain nervous pathway, μORs are located on synaptic terminals where they reduce the neurotransmitter release [35] , while somatic and dendritic receptors induce a strong hyperpolarization of the neuron. This may result from an inhibition of calcium channels or from a direct effect on the release machinery downstream from the calcium entry, as well as from membrane hyperpolarization through the activation of K + channels [36] , [37] . Similarly to μOR, the TREK-1 channel is located both in pre- and post-synaptic compartments of the central nervous system [38] , [39] , [40] . Thus, TREK-1 disinhibition by morphine through the activation of μOR may take place at the presynaptic afferences where it would limit the excitatory neurotransmitter release. Or, on the other hand, activation of postsynaptic TREK-1 channels may participate in the morphine-induced inhibition of secondary projection neurons. The hyperpolarization caused by TREK-1 opening might increase the voltage-dependent Mg 2+ blockade of NMDA receptors [39] and therefore reduce neurotransmission [41] . TREK-1 could therefore participate in the spinal inhibitory effect of morphine on pain transmission, in combination with GIRK channels, located at the postsynaptic level [42] , [43] . Tolerance to the analgesic effect of morphine implies that the amount of drug required to elicit pain relief must be increased to maintain analgesia. Opioid tolerance is usually associated with a decrease in opioid receptor sensitivity and expression in the plasma membrane, and with alterations of signalling mechanisms. It has been proposed that chronic exposure to morphine tonically enhances the cAMP pathway via the superactivation of adenylate cyclase and alters gene expression through the cAMP-responsive element-binding protein phosphorylation and expression [44] , [45] . The cAMP/PKA pathway inhibits the TREK-1 channel [27] , and therefore chronic exposure to morphine could lead to constitutive TREK-1 inhibition. Considering the role that we observe for TREK-1 in morphine analgesia, inhibition of TREK-1 could explain the tolerance to the analgesic effect of low doses of morphine and the reduction in tolerance to these doses in TREK-1 KO mice compared with their wild-type littermates. This reinforces the idea of an important contribution of the TREK-1 channel in the antinociceptive and antihyperalgesic effects of morphine and confirms that the TREK-1 channel can be considered as a downstream effector of μOR involved in the opioid-induced analgesia. However, the reduced influence of TREK-1 in analgesia and especially in tolerance induced by high doses of morphine, shown in KO mice, suggests that other effectors than TREK-1 could be involved, which is in line with previous studies suggesting an involvement of GIRK channels for these doses [16] , [17] . Morphine induces several adverse effects in humans as well as in rodents. At analgesic doses, the inhibition of gastrointestinal transit occurs, and constipation is a recurring complaint among patients under prolonged opioid treatment. This has motivated recent innovative therapeutic approaches to reduce it [46] . Interestingly, contrary to its antinociceptive effect, morphine-induced reduction in gastroinstestinal tract function was unchanged in TREK-1 KO mice; all parameters tested were identical in both genotypes. This result is consistent with the recent observations that the nitrergic-induced inhibition of neuromuscular transmission in the gastrointestinal tract, an important factor in morphine-induced constipation [47] , does not involve TREK-1 channels [48] . It demonstrates that analgesia and constipation, two usual effects of opioids, do not involve the same mechanisms downstream from μOR. Therefore, they may be dissociated. This is a very important finding because of the high prevalence of constipation in patients treated with opioids [49] , and the observation that for some patients in advanced illness opioid-induced constipation can rival distress caused by pain [50] . At higher doses, morphine induces a decrease in respiratory frequency, and this can have critical consequences, especially in the case of overdose [51] or in patients with respiratory failure [52] . Opioids induce respiratory depression by a number of mechanisms and neuronal sites of action [53] , including the pre-Botzinger complex of the ventrolateral medulla, which makes this effect mechanistically complex. Again, contrary to its antinociceptive effect, morphine-induced decrease in the respiratory rate was unchanged in TREK-1 KO mice, excluding the involvement of this channel in this adverse opioid effect. Chronic exposure to morphine also leads to dependence, which is apparent through the withdrawal syndrome triggered by the abrupt discontinuation of morphine exposure. Although correlations have been described between tolerance and dependence [54] , [55] , evidence of independent mechanisms between these two phenomenon also exists [56] . Our present work demonstrates, for all the symptoms explored, that the TREK-1 channel is not involved in the naloxone-induced withdrawal syndrome to chronic exposure to morphine. This observation, together with a recent work showing only a very modest contribution of all TREK channels in opioid-induced reward-related behaviour [57] , excludes the TREK-1 channel from a role in morphine-induced dependence and distinguishes it from GIRK channels that have clearly been involved in this effect of morphine. Indeed, Cruz et al. [17] have demonstrated that GIRK channels, possibly via the postsynaptic inhibition of the adrenergic neurons of the locus coeruleus, constitute an inhibitory gate for the induction of dependence. Taken together, our results show for the first time that there is a major involvement of the TREK-1 channel in the analgesic effect of μOR agonists both in acute nociceptive and painful pathological conditions and that this channel is not involved in the usual adverse effects of acute or chronic exposure to morphine such as constipation, respiratory depression and dependence. This demonstrates that analgesic and some of the most common adverse effects of morphine are mediated by different effectors downstream from μOR. Acting downstream μOR, directly on the TREK-1 channel, would be expected to provide an opportunity to dissociate the analgesic from the major adverse effects of opioids for pain therapies. Therefore, the TREK-1 channel could be a target of choice to design novel analgesic compounds as effective as morphine but devoid of its main adverse effects, which could be a major progress in the pharmacological therapy of pain. However, validation of this concept needs to perform studies with specific TREK-1 activators and it would be interesting to determine the lack of depressive effect of these compounds because of the antidepressant phenotype of TREK-1 KO mice [58] . Animals TREK-1 −/− mice have been generated by homologous recombination leading to the deletion of exon 3, which encodes the TM1 domain of the channel [41] . Heterozygous TREK-1-deficient mice were then backcrossed with C57Bl/6J congenic mice (Charles River, France) over 10 generations. All animals ( TREK-1 +/+ and TREK-1 −/− ) were 8- to 12-week-old males of N6F2 to N10F2 backcross generation. Mice were housed in grouped cages in a temperature-controlled environment with food and water ad libitum . The behavioural experiments were performed blind to the genotype and to the treatment, in a quiet room, by the same experimenter for a given test, and taking great care to avoid or minimize discomfort of the animals. All animal procedures were approved by the local Animal Ethics Committee (Comité d’Ethique en matière d’Expérimentation Animale en Auvergne, CEEA-02, France) and experiments were performed according to the guidelines provided by the European Community guiding in the care and use of animals (86/609/CEE). Drugs The following drugs were used: morphine hydrochloride (1–50 mg kg −1 for in vivo experiment and 1 μM for in vitro experiments) (Cooper, Melun, France), fentanyl (0.03 mg kg −1 ), naloxone hydrochloride (2 mg kg −1 ), tertiapine (30 pmol) and methylene blue (1 mg ml −1 ) (Sigma-Aldrich Chimie S.a.r.l., Lyon, France). All drugs were prepared just before use in 0.9% (w/v) NaCl solution, except for methylene blue dissolved in a 10% dextrose solution. Behavioural assessment of analgesic effect of morphine Several experimental series were performed: the first one to comparatively determine the kinetics (15, 30, 45, 60 and 90 min after treatment) of the effect of morphine in healthy WT and KO mice using two tests of thermal nociception (the heated water immersion assay and the hot-plate test); the second one to establish the ED50 of morphine in both genotypes at the peak effect (30 min after treatment); and the last one to determine kinetics in neuropathic and post-surgical pain models. For the heat water immersion assay, water temperature was kept constant at 46.0±0.2 °C using a thermoregulated water bath. Mice were maintained under a soft cloth except their tail/left hindpaw, which was immersed in water until withdrawal was observed (cutoff time of 40 s) [59] . For the hot-plate test, mice were placed on the plate (52.0±0.2 °C) and latencies to the first response characterized by the following signs were assessed: licking, shaking hindpaws or jumping (cutoff time of 40 s) [60] . Unilateral peripheral mononeuropathy was induced in mice anaesthetized with sodium pentobarbital (60 mg kg −1 , i.p.) with three chromic gut (4-0) ligatures tied loosely (with about 1-mm spacing) around the common sciatic nerve [25] . The nerve was constricted to a barely discernable degree, so that circulation through the epineurial vasculature was not interrupted. Heat sensitivity was tested 14 days after surgery by immersing the ipsilateral hindpaw to the partial nerve ligature of gently restrained mice in a water bath at 46 °C. The plantar incisional pain model was operated as initially described by Brennan et al. [24] Mice were anaesthetized with isoflurane 2.5%, and the skin of the operated foot was cleaned with povidone iodine 10% (Merck) and placed in the hole of a sterile drape. A 5-mm longitudinal incision was made through the skin and the fascia of plantar face of the left hindpaw, starting at 2 mm from the proximal edge of the heel. The plantar muscle was then incised longitudinally keeping attention to leave muscle origins intact. Behavioural pain test was performed 48 h after surgery by immersing the ipsilateral hindpaw to the surgery of gently restrained mice in a water bath at 46 °C. Naloxone-precipitated withdrawal syndrome Animals were first given twice daily morphine injections (10 mg kg −1 s.c.) for 6 days (and one final injection on day 7) [61] . Withdrawal was precipitated on day 7 by injecting naloxone (2 mg kg −1 , i.p.) 2 h after the final administration of morphine [62] . Ten minutes before naloxone treatment, mice were placed in a transparent acrylic box (20 cm in diameter, 60 cm high) to habituate to the new environment. Immediately after naloxone challenge, each mouse was placed back in the box gently, and the frequency of naloxone-precipitated withdrawal signs (escape jumps, teeth chattering, paw tremour) was recorded for 30 min. These symptoms were only seen following withdrawal. We have performed additional experiments by submitting wild-type mice to a 6-day regimen of saline injections followed by naloxone injection (2 mg kg −1 , i.p.). We failed to see any signs of withdrawal in this case. Tolerance paradigm The tail immersion test was used to determine tolerance paradigm. On the first day, baselines (drug-free pain thresholds) were first established; then mice were tested 30 min after subcutaneous administration of 0, 1, 3 or 5 mg kg −1 morphine. From the next morning on, mice received two daily morphine injections (10 mg kg −1 s.c.) for 6 days (only one injection on day 7) [61] . Finally, on day 8, mice were re-tested using tail immersion as described for day 1. Comparison between day 1 and day 8 allowed evaluating the development of morphine tolerance. It is indicated by a significant decrease in analgesic effect of morphine on day 8 as compared with day 1. Assessment of respiratory effect of morphine Whole-body plethysmography was performed in a noninvasive manner [63] , [64] , using an eight-chamber barometric plethysmograph apparatus (Emka Technologies, VA, USA) allowing the simultaneous monitoring of several animals of each genotype in parallel. The integrated software analysis (IOX, Emka Technologies, VA, USA) was used for calculation of the respiratory frequency. Mice were habituated to the chamber for 15 min prior to injection. Analysis of respiratory frequency over the 15-min habituation period revealed that the last 5 min produced relatively steady respiratory frequency. Therefore, breathing rate in this period was used to normalize the drug-induced effects over the 1.5-h test period. Assessment of gastrointestinal effect of morphine Fecal boli accumulation was evaluated on mice that were housed together prior to the test and provided food and water ad libitum . To assure that both genotypes were similarly eating, food consumption was monitored (grams of food consumed in 24 h) and normalized per mouse. Mice were then treated with saline or morphine (1, 3 or 5 mg kg −1 , s.c.) and placed individually in Plexiglass boxes with a grid floor. Fecal boli were collected and weighed 2 h post-treatment. Gastrointestinal transit was evaluated on mice that have received an injection of 0.1 ml of methylene blue-labelled 10% dextrose solution, using oral gavage. Thirty minutes later, the mice were killed. The stomach was clamped with a string above the lower oesophageal sphincter and a string beneath the pylorus to prevent the leakage of methylene blue. The intestinal transit was measured from the pylorus to the most distal point of migration of methylene blue. It was expressed as the percentage of total intestinal length [65] , [66] . Colonic migrating motor complexes were measured as described by Fida et al. [67] The entire colon was removed and placed in a dish containing modified Kreb’s solution (see composition below) at 4 °C, flushed of faecal material and the mesentery was dissected away. A stainless steel, side-hole tube inserted through the lumen of the colon was used to secure the preparation into an organ bath that was continuously perfused with modified Kreb’s solution (3 ml min −1 ) containing (in mM) the following: NaCl 120, KCl 5, NaH 2 PO 4 -2H 2 O 1, MgSO 4 -7H 2 O 1, NaHCO 3 25, glucose 11 and CaCl 2 2.5, bubbled with 95% O 2 and 5% CO 2 and maintained at 36.0±0.5 °C. Three stainless steel hooks were inserted through the muscularis externa perpendicular to the long axis of the colon. The hooks were placed 1.5 cm apart and about 2 cm from each end of the colon. Each hook was hung up on a Grass FT03 isometric force transducer to record circular muscle contractions from the proximal, intermediate and distal parts of the colon, respectively. Tension, which was initially set to below 10 mN, was monitored continuously using an MP150 interface and was recorded on a PC running Acknowledge 3.7.2 software (BIOPAC systems, Santa Barbara, CA, USA). Electrophysiological experiments COS cells were plated at a density of 20,000 cells per 35-mm petri dish and grown at 37 °C in DMEM containing 10% of fetal bovine serum and 1% of antibiotics (penicillin and streptomycin). Transfections were performed using the JetPEI reagent 1 day after plating, according to the supplier’s protocol. Briefly, cells were incubated 4–6 h with a mix of pIRES2-muOR-EGFP, pIRES2-TREK-1-EGFP or the mutant pIRES2-TREK-1S333D-EYFP, and JetPEI (2 μl per μg of plasmids) [38] . TREK-1-S333D mutant is analogous to the phosphorylated form of TREK-1 thus to the PKA-mediated inhibited form of the channel. Transfected cells, identified by their green fluorescence, were used for whole-cell voltage-clamp recordings 2–4 days after transfection. We used the whole-cell voltage-clamp configuration of the patch-clamp technique to measure membrane currents from transfected COS-7 cells. Current levels were measured at 0 mV as the difference with current levels at –80 mV, the reversal potential for K+. In control experiments with COS cells transfected with μOR, there was no activation of endogenous currents by 10 μM morphine or 10 μM arachidonic acid ( n =4, P >0.1, Wilcoxon matched pairs test ( Supplementary Fig. S5 ). Recordings were made at room temperature using an axopatch 200B amplifier (Axon Instruments) with a 3-kHz low-pass filter (Krohn-Hite). Data were sampled at 10 kHz, digitized by a Digidata 1440 A-D/D-A converter (Axon Instruments) and recorded on a hard drive using the pClamp software (version 10, Axon Instruments). Patch pipettes (1–4 MΩ) contained (in mM) the following: 135 KCl, 5 NaCl, 2 MgCl 2 , 5 EGTA, 10 HEPES (pH 7.25 with KOH) and the control bath solution contained (in mM) the following: 145 NaCl, 5 KCl, 2 MgCl 2 , 2 CaCl 2 , 10 HEPES (pH 7.4 with NaOH). Drugs of interest were dissolved at their final concentration in the control bathing solution and were applied to individual patch-clamped cells using a home-made microperfusion system driven by microsolenoid valves (Sirai, Italy) allowing rapid solution changes. Statistical analysis Data, expressed as mean±s.e.m., were analysed using Sigma STAT Software version 3.0 for Windows (STAT32 Software Inc., San Diego, CA, USA). The specific tests used are indicated within the text of the figure legends. How to cite this article: Devilliers, M. et al. Activation of TREK-1 by morphine results in analgesia without adverse side effects. Nat. Commun. 4:2941 doi: 10.1038/ncomms3941 (2013).